Dynamic switching of calmodulin interactions underlies Ca2+regulation of CaV1.3 channels Calmodulin regulation of Ca V channels is a prominent Ca 2+ feedback mechanism orchestrating vital adjustments of Ca 2+ entry. The long-held structural correlation of this regulation has been Ca 2+ -bound calmodulin, complexed alone with an IQ domain on the channel carboxy terminus. Here, however, systematic alanine mutagenesis of the entire carboxyl tail of an L-type Ca V 1.3 channel casts doubt on this paradigm. To identify the actual molecular states underlying channel regulation, we develop a structure–function approach relating the strength of regulation to the affinity of underlying calmodulin/channel interactions, by a Langmuir relation (individually transformed Langmuir analysis). Accordingly, we uncover frank exchange of Ca 2+ –calmodulin to interfaces beyond the IQ domain, initiating substantial rearrangements of the calmodulin/channel complex. The N-lobe of Ca 2+ –calmodulin binds an N-terminal spatial Ca 2+ transforming element module on the channel amino terminus, whereas the C-lobe binds an EF-hand region upstream of the IQ domain. This system of structural plasticity furnishes a next-generation blueprint for Ca V channel modulation. Calmodulin (CaM) regulation of the Ca V 1–2 family of Ca 2+ channels ranks among the most consequential of biological Ca 2+ decoding systems [1] , [2] . In this regulation, the Ca 2+ -free form of CaM (apoCaM) already pre-associates with channels [3] , [4] , [5] , ready for ensuing Ca 2+ -driven modulation of channel opening. Upon elevation, intracellular Ca 2+ binds to this indwelling CaM, driving conformational changes that enhance opening in some channels [6] , [7] , [8] (positive-feedback ‘facilitation’) and inhibit opening in others [9] , [10] (negative-feedback ‘inactivation’). Intriguingly, Ca 2+ binding to the individual carboxy- and amino-terminal lobes of CaM can semiautonomously induce distinct components of channel regulation [7] , [9] , [11] , where the C-lobe responds well to Ca 2+ entering through the channel on which the corresponding CaM resides (‘local Ca 2+ selectivity’), and the N-lobe may, in some channels, require the far weaker Ca 2+ signal from distant Ca 2+ sources [6] , [7] , [12] , [13] , [14] (‘global Ca 2+ selectivity’). Such Ca 2+ -feedback regulation influences many biological functions [1] , [15] , [16] , [17] and furnishes mechanistic lessons for Ca 2+ decoding [14] . Indeed, CaM regulation of L-type (Ca V 1.2) channels strongly influences cardiac electrical stability [15] , [18] , and pharmacological manipulation of such regulation looms as a future antiarrhythmic strategy [18] , [19] . Crucial for understanding and manipulating this CaM regulatory system is the identification of the conformations that underlie such Ca 2+ modulation. 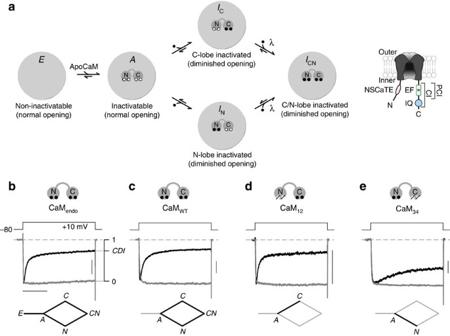Figure 1: General schema for CaM regulation of representative L-type CaV1.3 channels. (a) Primary configurations of CaM/channel complex with respect to CaM-regulatory phenomena (E,A,IC,INandICN). Inset at far right, cartoon of main channel landmarks involved in CaM regulation, with only the pore-formingα1Dsubunit of CaV1.3 diagrammed. Ca2+-inactivation (CI) region, in the proximal channel C terminus (~160 amino acids (aa)), contains elements potentially involved in CaM regulation. IQ domain (IQ), comprising the C-terminal ~30 aa of the CI segment, long proposed as preeminent for CaM/channel binding. Dual vestigial EF-hand (EF) motifs span the proximal ~100 aa of the CI module; these have been proposed to play a transduction role in channel regulation. Proximal CI (PCI) region constitutes the CI element exclusive of the IQ domain. NSCaTE on channel N terminus of CaV1.2–1.3 channels may be the N-lobe Ca2+/CaM effector site. (b) Whole-cell CaV1.3 currents expressed in HEK293 cell, demonstrating CDI in the presence of endogenous CaM only. CDI observed here can reflect properties of the entire system diagrammed ina, as schematized by the stick-figure diagram at the bottom ofb. Here and throughout, the vertical scale bar pertains to 0.2 nA of Ca2+current (black); and the Ba2+current (gray) has been scaled ~3-fold downward to aid comparison of decay kinetics, here and throughout. Horizonal scale bar, 100 ms. (c) Currents during overexpression of CaMWT, isolating the behaviour of the diamond-shaped subsystem at bottom. (d) Currents during overexpression of CaM12, isolating C-lobe form of CDI. (e) Currents during overexpression of CaM34, isolating N-lobe form of CDI. (c–e) Vertical bar, 0.2 nA Ca2+current. Timebase as inb. Figure 1a summarizes the currently accepted conceptual framework, with specific reference to L-type Ca V 1.3 channels for concreteness. Configuration E (‘empty’ of CaM) represents channels lacking preassociated apoCaM. Such channels can open normally, but do not exhibit Ca 2+ /CaM-dependent inactivation (CDI) over the typical ~300 ms duration of channel-activity measurements [20] . Over this period, Ca 2+ /CaM from the bulk solution cannot appreciably access a channel in configuration E to produce CDI [20] , [21] , [22] , [23] . ApoCaM preassociation with configuration E yields channels in configuration A , where opening can also proceed normally, but subsequent CDI can now ensue. A thereby denotes channels that are ‘active’ and capable of CDI. Switching between configurations E and A occurs slowly (>10 s of seconds [24] ), and almost exclusively involves apoCaM, because typical experiments only briefly activate Ca 2+ channels every 20–30 s. Thus, there is negligible exchange with configuration E during typical measurements of current. Regarding CDI, Ca 2+ binding to both lobes of CaM yields configuration I CN (both C- and N-lobes of CaM engaged towards CDI), corresponding to a fully inactivated channel with strongly reduced opening [2] , [25] . As for intermediate configurations [7] , [9] , [11] , [14] , [26] , Ca 2+ binding only to the C-lobe induces configuration I C , representing a C-lobe inactivated channel with reduced opening; Ca 2+ binding only to the N-lobe yields an analogous N-lobe-inactivated configuration ( I N ), also with reduced opening. Subsequent entry into configuration I CN likely involves cooperative interactions denoted by a λ symbol. Overall, CDI reflects redistribution from configuration A into I C , I N and I CN . Of note, we exclude cases where one Ca 2+ binds a lobe of CaM, because binding within lobes is highly cooperative [27] . Moreover, only one CaM is included, based on multiple lines of evidence [22] , [23] . Figure 1: General schema for CaM regulation of representative L-type Ca V 1.3 channels. ( a ) Primary configurations of CaM/channel complex with respect to CaM-regulatory phenomena ( E , A , I C , I N and I CN ). Inset at far right, cartoon of main channel landmarks involved in CaM regulation, with only the pore-forming α 1D subunit of Ca V 1.3 diagrammed. Ca 2+ - i nactivation (CI) region, in the proximal channel C terminus (~160 amino acids (aa)), contains elements potentially involved in CaM regulation. IQ domain (IQ), comprising the C-terminal ~30 aa of the CI segment, long proposed as preeminent for CaM/channel binding. Dual vestigial EF-hand (EF) motifs span the proximal ~100 aa of the CI module; these have been proposed to play a transduction role in channel regulation. Proximal CI (PCI) region constitutes the CI element exclusive of the IQ domain. NSCaTE on channel N terminus of Ca V 1.2–1.3 channels may be the N-lobe Ca 2+ /CaM effector site. ( b ) Whole-cell Ca V 1.3 currents expressed in HEK293 cell, demonstrating CDI in the presence of endogenous CaM only. CDI observed here can reflect properties of the entire system diagrammed in a , as schematized by the stick-figure diagram at the bottom of b . Here and throughout, the vertical scale bar pertains to 0.2 nA of Ca 2+ current (black); and the Ba 2+ current (gray) has been scaled ~3-fold downward to aid comparison of decay kinetics, here and throughout. Horizonal scale bar, 100 ms. ( c ) Currents during overexpression of CaM WT , isolating the behaviour of the diamond-shaped subsystem at bottom. ( d ) Currents during overexpression of CaM 12 , isolating C-lobe form of CDI. ( e ) Currents during overexpression of CaM 34 , isolating N-lobe form of CDI. ( c – e ) Vertical bar, 0.2 nA Ca 2+ current. Timebase as in b . Full size image The structural basis of this conceptual foundation is less certain, but has been dominated by an IQ-centric hypothesis, where an IQ domain, present on the C termini of all Ca V 1–2 channels [2] ( Fig. 1a , far right, blue circle), serves as the dominant CaM-binding locus on the channel. By this hypothesis, not only does this element comprise much of the preassociation surface for apoCaM [4] , [5] , [20] ( Fig. 1a , configuration A ), it also constitutes the primary effector site [2] , [5] , [7] , [9] , [10] , [25] , [28] for Ca 2+ /CaM rebinding to induce Ca 2+ regulation (for example, Fig. 1a , I CN ). The predominance of the IQ-centric paradigm [2] has prompted resolution of several crystal structures of Ca 2+ /CaM complexed with IQ-domain peptides of various Ca V 1–2 channels [29] , [30] , [31] , [32] . Nonetheless, certain findings fit poorly with this viewpoint. First, crystal structures of Ca 2+ /CaM complexed with wild-type (WT) and mutant IQ peptides of Ca V 1.2 indicate that a signature isoleucine in the IQ element is deeply buried within the C-lobe of Ca 2+ /CaM, and that alanine substitution at this isoleucine negligibly perturbs structure [30] . Moreover, Ca 2+ /CaM affinities for analogous WT and mutant IQ peptides are nearly identical [28] . How then does alanine substitution at this well-encapsulated locus influence the rest of the channel to strongly disrupt functional regulation [30] ? Second, in Ca V 1.2/1.3 channels we have demonstrated that the effector interface for the N-lobe of Ca 2+ /CaM resides within an N-terminal spatial Ca 2+ transforming element (NSCaTE) element of the channel N terminus [13] , [14] , [33] ( Fig. 1a , far right), separate from the IQ element. Third, analysis of the atomic structure of Ca 2+ /CaM bound to an IQ peptide of Ca V 2.1 channels hints that the C-lobe effector site also resides somewhere outside the IQ module [31] . In all, the long disconnect between challenges like these and IQ-centric theory represents a critical impasse in the field. A major concern with prior IQ-domain analyses is that function was mostly characterized with only endogenous CaM present [5] , [10] , [25] , [28] , [31] . This regime is problematic, as IQ-domain mutations could alter CaM regulation via perturbations at multiple steps within Fig. 1a , whereas interpretations mainly ascribe effects to altered Ca 2+ /CaM binding with an IQ effector site. Serious interpretive challenges thus include the following: (1) although the high apoCaM affinity of most WT channels [4] , [20] renders configuration E unlikely ( Fig. 1a ), this may not hold true for mutant channels, just as observed for certain Ca V 1.3 splice variants [20] . Mutations weakening apoCaM preassociation could thereby reduce CDI by favouring configuration E ( Fig. 1a , incapable of CDI), without affecting Ca 2+ /CaM binding. (2) Mutations that do weaken interaction with one lobe of Ca 2+ /CaM may have their functional effects masked by cooperative steps ( λ in Fig. 1a ). This study systematically investigates the IQ-centric hypothesis, minimizing the above challenges by focusing on Ca V 1.3 channels, a representative L-type channel whose CDI is particularly robust and separable into distinct C- and N-lobe components [11] , [13] , [14] . These attributes simplify analysis as follows. For orientation, Fig. 1b illustrates the CDI of Ca V 1.3 channels expressed in HEK293 cells, with only endogenous CaM present. Strong CDI is evident from the rapid decay of whole-cell Ca 2+ current (black trace) compared with the nearly absent decline of Ba 2+ current (gray trace). As Ba 2+ binds negligibly to CaM [34] , the fractional decline of Ca 2+ versus Ba 2+ current after 300 ms depolarization quantifies the steady-state extent of CDI ( Fig. 1b , right, CDI parameter). The CDI here reflects the operation of the entire Fig. 1a system, as schematized at the bottom of Fig. 1b . We can formally isolate the diamond-shaped subsystem lacking configuration E ( Fig. 1c , bottom), by using mass action and strong overexpression of WT CaM (CaM WT ). The resulting CDI ( Fig. 1c ) is indistinguishable from that with only endogenous CaM present ( Fig. 1b ), owing to the high apoCaM affinity of WT Ca V 1.3 channels. Full deconstruction of CDI arises upon strong coexpression of channels with a mutant CaM that only allows Ca 2+ binding to its C-terminal lobe [9] ( Fig. 1d , CaM 12 ). With reference to Fig. 1a , this manoeuvre depopulates configuration E by mass action, and forbids access into configurations I N and I CN . Thus, the isolated C-lobe component of CDI [11] , [14] is resolved ( Fig. 1d ), with its signature rapid timecourse of current decay. Importantly, this regime avoids interplay with cooperative λ steps in Fig. 1a . Likewise, strongly coexpressing mutant CaM exhibiting Ca 2+ binding to its N-lobe alone [9] (CaM 34 ) isolates the slower N-lobe form of CDI [11] , [14] ( Fig. 1e ), with attendant simplifications. Thus armed, we here exploit selective monitoring of Ca V 1.3 subsystems ( Fig. 1b–e ), combined with alanine, scanning mutagenesis of the entire carboxyl tail of Ca V 1.3 channels. In doing so, we argue against the IQ-centric paradigm and propose a new framework for the CaM regulation of Ca 2+ channels. Individually transformed Langmuir analysis of CaM/channel regulation Identifying channel effector interfaces for Ca 2+ /CaM is challenging. The main subunit of Ca V channels alone spans about 2,000 amino acids or more; and peptide assays indicate that Ca 2+ /CaM can bind to multiple segments of uncertain function [25] , [35] , [36] , [37] , [38] , [39] . Even if mutating these segments alters CaM regulation, the observed functional effects could reflect perturbations of apoCaM preassociation, Ca 2+ /CaM binding or transduction. To address these challenges, we initially consider an expanded conceptual layout believed valid for either isolated N- or C-lobe CDI [14] ( Fig. 2a ), then deduce from this arrangement a simple quantitative analysis to identify bona fide effector interfaces. An apoCaM lobe begins prebound to a channel preassociation surface (state 1). Ca 2+ binding to CaM in this prebound state is considered rare [14] , [40] . However, after apoCaM releases (state 2), it may bind Ca 2+ to produce Ca 2+ /CaM (state 3), or return to state 1. The transiently dissociated lobe of CaM (state 2 or 3) remains within a channel alcove over the usual timescale of CaM regulation (≤seconds). Finally, Ca 2+ /CaM binds a channel effector site (state 4, square pocket), ultimately inducing regulation via transduction to state 5. Emergent behaviours of this scheme rationalize local and global Ca 2+ selectivities, as argued previously [14] . 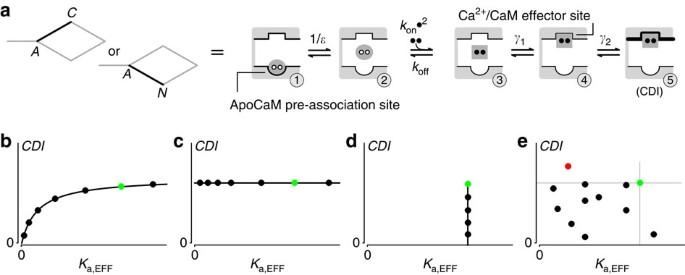Figure 2: Probing functionally relevant CaM regulatory interactions via iTL analysis. (a) Isolated C- or N-lobe regulatory system (denoted by stick-figure diagrams on left) can be coarsely represented by a five-state scheme on right. A single lobe of apoCaM begins preassociated to channel (state 1). Following disassociation (state 2), CaM may bind two Ca2+ions (state 3, black dots). Ca2+/CaM may subsequently bind to channel effector site (state 4). From here, transduction step leads to state 5, equivalent to CDI. Association constant for lobe of apoCaM binding to preassociation site isε; whereasγ1andγ2are association constants for respective transitions from states 3 to 4, and states 4 to 5. (b) Unique Langmuir relation (equation 1) that will emerge upon plotting channelCDI(definedFig. 1b, right) as a function ofKa,EFF(association constant measured for isolated channel peptide), ifKa,EFFis proportional to one of the actual association constants in the scheme as ina. Black symbols, hypothetical results for various channel/peptide mutations; green symbol, hypothetical WT. (c) Predicted outcome if peptide association constantKa,EFFhas no bearing on association constants within holochannels. (d) Outcome if mutations affect holochannel association constants, but not peptide association constants. (e) Outcome if mutations affect holochannel association constant(s) and peptide association constant, but in ways that are poorly correlated. Figure 2: Probing functionally relevant CaM regulatory interactions via iTL analysis. ( a ) Isolated C- or N-lobe regulatory system (denoted by stick-figure diagrams on left) can be coarsely represented by a five-state scheme on right. A single lobe of apoCaM begins preassociated to channel (state 1). Following disassociation (state 2), CaM may bind two Ca 2+ ions (state 3, black dots). Ca 2+ /CaM may subsequently bind to channel effector site (state 4). From here, transduction step leads to state 5, equivalent to CDI. Association constant for lobe of apoCaM binding to preassociation site is ε ; whereas γ 1 and γ 2 are association constants for respective transitions from states 3 to 4, and states 4 to 5. ( b ) Unique Langmuir relation (equation 1) that will emerge upon plotting channel CDI (defined Fig. 1b , right) as a function of K a,EFF (association constant measured for isolated channel peptide), if K a,EFF is proportional to one of the actual association constants in the scheme as in a . Black symbols, hypothetical results for various channel/peptide mutations; green symbol, hypothetical WT. ( c ) Predicted outcome if peptide association constant K a,EFF has no bearing on association constants within holochannels. ( d ) Outcome if mutations affect holochannel association constants, but not peptide association constants. ( e ) Outcome if mutations affect holochannel association constant(s) and peptide association constant, but in ways that are poorly correlated. Full size image Despite the multiple transitions present even for this reduced CDI subsystem ( Fig. 2a , left schematics), a straightforward relationship emerges that will aid detection of Ca 2+ /CaM interfaces on the channel, as follows. Suppose we can introduce point alanine mutations into the channel that selectively perturb the Ca 2+ /CaM-binding equilibrium association constant γ 1 ( Fig. 2a ). Moreover, suppose we can measure Ca 2+ /CaM binding to a corresponding channel peptide, and the affiliated association constant ϰ a,EFF is proportional to γ 1 in the channel. It then turns out that our metric of inactivation ( CDI in Fig. 1b ) will always be given by the Langmuir function where CDI max is the value of CDI if ϰ a,EFF becomes exceedingly large, and Λ is a constant comprised of other association constants in the layout ( Supplementary Note S1 ). Figure 2b plots this function, where the green symbol marks a hypothetical WT channel position, and mutations should create data symbols that decorate the remainder of the curve. Importantly, the requirement that peptide K a,EFF need only be proportional to (not equal to) holochannel γ 1 increases the chances that tagged peptides may suffice to correlate with holochannel function. In addition, equation 1 will hold true only if these two suppositions are satisfied ( Supplementary Note S2 ). For example, if mutations alter two transitions within the holochannel, a function with different shape will result. Alternatively, if mutations change the peptide interaction with Ca 2+ /CaM ( ϰ a,EFF ), but not any of the actual association constants within the channel, the outcome in Fig. 2c will emerge. In this case, though the channel peptide can bind Ca 2+ /CaM in isolation, this reaction has no bearing on transitions within the intact holochannel ( Fig. 2a ). By contrast, Fig. 2d diagrams a scenario where mutations actually do affect transition(s) governing CDI within the holochannel, yet altogether fail to perturb Ca 2+ /CaM binding to a peptide segment of the channel. It is also possible that mutations could affect transition(s) governing CDI within the holochannel, but in ways that are uncorrelated with mutational perturbations of Ca 2+ /CaM binding to a corresponding peptide segment ( Fig. 2e ). The red symbol denotes a specific subset of this scenario, where a mutation affects transition(s) within the holochannel so as to enhance CDI, whereas the same mutation produces uncorrelated diminution of Ca 2+ /CaM binding to a peptide segment of the channel. Yet other deviations from equation 1 are possible, including those arising from the existence of effector sites beyond our alanine scan ( Supplementary Note S3 ). Importantly, these outcomes will pertain, regardless the size and complexity of the scheme in Fig. 2a ( Supplementary Note S4 ). Because of this generality, we term the analysis individually transformed Langmuir (iTL) analysis. Given this insight, we undertook alanine-scanning mutagenesis of Ca V 1.3 channel domains, and screened electrophysiologically for altered CaM regulatory hotspots. In parallel, we introduced hotspot mutations into peptides overlapping scanned regions, and estimated K a,EFF of potential CaM binding. For this purpose, we utilized live-cell fluorescence resonance energy transfer (FRET) two-hybrid assays [3] , [4] , [41] , which have the resolution and throughput for the task. If such binding truly reflects holochannel function, then CDI should vary with K a,EFF as a Langmuir function (equation 1, Fig. 2b ). By contrast, if K a,EFF changes in a manner unrelated to holochannel CDI, data would diverge from equation 1 ( Fig. 2c–e , or otherwise). CaM effector interfaces could thus be systematically resolved. iTL analysis of IQ domain as Ca 2+ /CaM effector site We first addressed whether the Ca V 1.3 IQ domain serves as a Ca 2+ /CaM effector site for CDI, as IQ-centric theory postulates. Single alanines were substituted at each position of the entire IQ domain of Ca V 1.3 channels, whose sequence appears atop Fig. 3a , with the signature isoleucine bolded at position ‘0’. Naturally occurring alanines were changed to threonine. CDI of these mutants was then characterized for the isolated N- and C-lobe CDI subsystems described above ( Fig. 3a , left schematics), thus minimizing potential complications from diminished preassociation with apoCaM ( Fig. 1a , configuration E ), or masking of CDI effects by cooperative λ steps ( Fig. 1a ). Whereas little deficit in N-lobe CDI was observed ( Fig. 3a ), the C-lobe CDI was strongly attenuated by alanine substitutions at I[0]A ( Fig. 3b , red bar, exemplar traces) and nearby positions (rose). To test for correspondence between reductions in C-lobe CDI and altered Ca 2+ /CaM binding, we performed FRET two-hybrid assays of Ca 2+ /CaM binding to alanine-substituted IQ peptides, with substitutions encompassing sites associated with the strongest CDI effects ( Fig. 3b , red and rose bars). Hatched bars denote additional sites chosen at random. The left aspect of Fig. 3c cartoons the FRET interaction partners, and the right portion displays the resulting binding curve for the WT IQ peptide ( Fig. 3c , right, black). FR -1 is proportional to FRET efficiency, as indicated by the efficiency E A scale bar on the right. D free is the free concentration of donor-tagged molecules (cyan fluorescent protein (CFP)–CaM), where 200 nM is approximately 6,100 D free units [4] , [42] . At odds with a Ca 2+ /CaM effector role of the IQ domain, the binding curve for the I[0]A substitution ( Fig. 3c , right, red) resembled that for the WT peptide (black), whereas C-lobe CDI was strongly decreased ( Fig. 3b ). 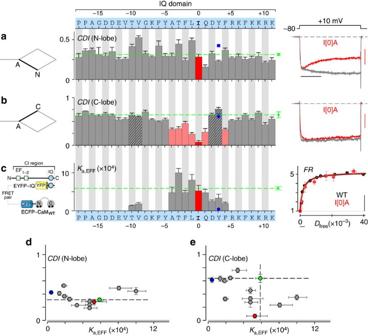Figure 3: Inconsistencies with IQ domain role as Ca2+/CaM effector site. (a) No appreciable deficit in isolated N-lobe CDI upon point alanine substitutions across the IQ domain (sequence at top with bolded isoleucine at ‘0’ position). Left, corresponding subsystem schematic. Middle, bar-graph summary ofCDImetric, as defined inFig. 1b. Bars, mean±s.e.m. for ~6 cells each. Green dashed line, WT profile; red bar, I[0]A; blue symbol in all panels, Y[3]D. Right, exemplar currents, demonstrating no change in N-lobe CDI upon I[0]A substitution. Horizontal scale bar, 100 ms; vertical scale bar, 0.2 nA Ca2+current. Red, Ca2+current; gray, Ba2+current. (b) Isolated C-lobe CDI (corresponding subsystem schematized on left) exhibits significant attenuation by mutations surrounding the central isoleucine (coloured bars). Format as ina. I[0]A shows the strongest attenuation (red bar and exemplar currents at right). Bars average ~5 cells±s.e.m. Dashed green line, WT profile. Timebase as inb; vertical scale bar, 0.2 nA Ca2+current. (c) Bar-graph summary of association constants (Ka,EFF=1/Kd,EFF) for Ca2+/CaM binding to IQ, evaluated for constructs exhibiting significant effects inb(coloured bars, with I[0]A in red), or chosen at random (hashed inb). Error bars, non-linear s.d. estimates. FRET partners schematized on the left, and exemplar binding curves on the right for I[0]A (red) and WT (black). Symbols average ~7 cells. Smooth curve fits, 1:1 binding model. Calibration to efficiencyEA=0.1, far right vertical scale bar. Horizontal scale bar corresponds to 100 nM. (d) Plots of N-lobeCDIversusKa,EFFdeviate from equation 1, much as inFig. 2c. Green, WT; red, I[0]A; blue, Y[3]D. (e) Plots of C-lobeCDIversusKa,EFFalso diverge from Langmuir, as inFig. 1e. This result further argues against the IQper seacting as an effector site for the C-lobe of Ca2+/CaM. Symbols as ind. (d,e) Y[3]D (blue symbol,CDImean of four cells) yields poor Ca2+/CaM binding, but unchanged CDI.Supplementary Note S7, further FRET data. Figure 3c (middle) displays a bar-graph summary of the resulting association constants ( K a,EFF ); the WT value is shown as a dashed green line, and that for I[0]A as a red bar ( Supplementary Note S5 ). If the IQ domain were the effector site for the C-lobe of Ca 2+ /CaM, C-lobe CDI over various substitutions should correlate with association constants according to equation 1 ( Supplementary Notes S1 and S6 ). However, plots of our data markedly deviate from such a relation ( Fig. 3e ), much as in Fig. 2e . The green symbol denotes the WT IQ case. Likewise, plots of N-lobe CDI versus K a,EFF deviated from a Langmuir ( Fig. 3d ), much as in Fig. 2c . These outcomes fail to support the IQ domain as an effector site for either lobe of Ca 2+ /CaM. The actual role of the IQ domain in CDI will be explored later in Fig. 6. Figure 3: Inconsistencies with IQ domain role as Ca 2+ /CaM effector site. ( a ) No appreciable deficit in isolated N-lobe CDI upon point alanine substitutions across the IQ domain (sequence at top with bolded isoleucine at ‘0’ position). Left, corresponding subsystem schematic. Middle, bar-graph summary of CDI metric, as defined in Fig. 1b . Bars, mean±s.e.m. for ~6 cells each. Green dashed line, WT profile; red bar, I[0]A; blue symbol in all panels, Y[3]D. Right, exemplar currents, demonstrating no change in N-lobe CDI upon I[0]A substitution. Horizontal scale bar, 100 ms; vertical scale bar, 0.2 nA Ca 2+ current. Red, Ca 2+ current; gray, Ba 2+ current. ( b ) Isolated C-lobe CDI (corresponding subsystem schematized on left) exhibits significant attenuation by mutations surrounding the central isoleucine (coloured bars). Format as in a . I[0]A shows the strongest attenuation (red bar and exemplar currents at right). Bars average ~5 cells±s.e.m. Dashed green line, WT profile. Timebase as in b ; vertical scale bar, 0.2 nA Ca 2+ current. ( c ) Bar-graph summary of association constants ( K a,EFF =1/ K d,EFF ) for Ca 2+ /CaM binding to IQ, evaluated for constructs exhibiting significant effects in b (coloured bars, with I[0]A in red), or chosen at random (hashed in b ). Error bars, non-linear s.d. estimates. FRET partners schematized on the left, and exemplar binding curves on the right for I[0]A (red) and WT (black). Symbols average ~7 cells. Smooth curve fits, 1:1 binding model. Calibration to efficiency E A =0.1, far right vertical scale bar. Horizontal scale bar corresponds to 100 nM. ( d ) Plots of N-lobe CDI versus K a,EFF deviate from equation 1, much as in Fig. 2c . Green, WT; red, I[0]A; blue, Y[3]D. ( e ) Plots of C-lobe CDI versus K a,EFF also diverge from Langmuir, as in Fig. 1e . This result further argues against the IQ per se acting as an effector site for the C-lobe of Ca 2+ /CaM. Symbols as in d . ( d , e ) Y[3]D (blue symbol, CDI mean of four cells) yields poor Ca 2+ /CaM binding, but unchanged CDI. Supplementary Note S7 , further FRET data. Full size image To undertake a still more stringent test, we investigated a Y[3]D construct, based on a prior analogous mutation in Ca V 2.1 that intensely diminished Ca 2+ /CaM affinity [31] . Indeed, the Y[3]D substitution in Ca V 1.3 resulted in a large 13.5-fold decrement in K a,EFF ( Fig. 3c , blue symbol). However, there was no change in C- or N-lobe CDI ( Fig. 3a , blue symbols; Supplementary Note S7 ). These data deviated yet more strongly from a Langmuir (blue symbols, Fig. 3d ), arguing further against the IQ domain as a Ca 2+ /CaM effector site. NSCaTE element upheld as effector site for N-lobe of Ca 2+ /CaM Given the absence of a positive outcome for iTL analysis of the IQ domain (that is, Fig. 2b ), we turned to the N-terminal NSCaTE module ( Fig. 4a , oval), previously proposed as an effector site for N-lobe CDI [13] , [14] . For reference, Fig. 4b displays the WT Ca V 1.3 profile for N-lobe CDI. Single alanines were substituted across the NSCaTE module ( Fig. 4d , top), at residues that were not originally alanine. The bar-graph summary below ( Fig. 4d ) indicates strongly diminished N-lobe CDI upon alanine substitution at three residues, previously identified as critical [13] , [14] (W[44]A, I[48]A and R[52]A). For comparison, the WT level of CDI is represented by the green dashed line and affiliated error bars. W[44]A featured the strongest CDI decrement, as shown by the Ca 2+ current ( Fig. 4b , red trace) and population data ( Fig. 4d , red bar). To pursue iTL analysis, we characterized corresponding binding curves between NSCaTE and Ca 2+ /CaM 34 FRET pairs ( Fig. 4c , left; Supplementary Note S8 ). The WT pairing exhibited a well-resolved binding curve with K a,EFF =4 × 10 −4 D free −1 units ( Fig. 4c , right, black), whereas the W[44]A variant yielded a far lower affinity with K a,EFF ~0 (red). A summary of binding affinities is shown for this and additional mutations within NSCaTE in Fig. 4e ( Supplementary Note S9 ), where the dashed green line signifies the WT profile. The crucial test arises by plotting N-lobe CDI as a function of K a,EFF , which resolves the Langmuir relation in Fig. 4f . For reference, WT is shown in green and W[44]A in red. The particular formulation of equation 1 for this arrangement is given in Supplementary Note S1 . Hence, iTL analysis does uphold NSCaTE as a predominate effector site for N-lobe CDI, as argued before by other means [13] , [14] . By contrast, analysis of C-lobe CDI ( Fig. 4g–k and Supplementary Note S10 ) reveals deviation from equation 1 ( Fig. 4l ), much as in Fig. 2c . Thus, NSCaTE mutations have little bearing on C-lobe CDI of the holochannel, though such mutations affect Ca 2+ /CaM 12 binding to an isolated NSCaTE peptide. 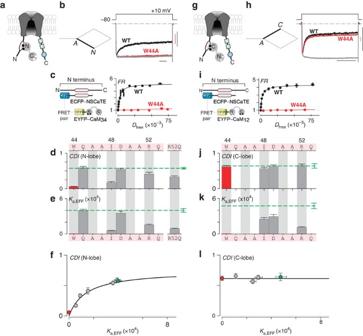Figure 4: iTL analysis of Ca2+/CaM effector role of NSCaTE module of CaV1.3 channels. (a) Cartoon depicting NSCaTE as putative effector interface for N-lobe of Ca2+/CaM. (b) Exemplar CaV1.3 whole-cell currents exhibiting robust isolated N-lobe CDI, as seen from the rapid decay of Ca2+current (black trace). Corresponding stick-figure subsystem appears on the left. W[44]A mutation abolishes N-lobe CDI, as seen from the lack of appreciable Ca2+current decay (red trace). Gray trace, averaged Ba2+trace for WT and W[44]A constructs. Horizontal scale bar, 100 ms; vertical scale bar, 0.2 nA Ca2+current (red, W44A; black, WT). (c) FRET two-hybrid binding curves for Ca2+/CaM34and NSCaTE segment, with FRET partners schematized on the left. WT pairing in black; W[44]A mutant pairing in red. Each symbol, mean±s.e.m. of ~5 cells. (d) Bar-graph summary of N-lobeCDIfor NSCaTE mutations measured after 800 ms depolarization, with NSCaTE sequence at the top, as numbered by position within CaV1.3. Data for W[44]A in red; dashed green line, WT. Bars, mean±s.e.m. of ~5 cells. (e) Association constants (Ka,EFF=1/Kd,EFF) for Ca2+/CaM34binding to NSCaTE module evaluated for constructs exhibiting significant effects in paneld. Error bars, non-linear s.d. estimates. Data for W[44]A in red; dashed green line, WT. (f) Plotting N-lobeCDIversusKa,EFFuncovers a Langmuir, identifying NSCaTE as functionally relevant effector site. W[44]A in red; WT in green. (g–l) iTL fails to uphold NSCaTE as effector site for C-lobe of Ca2+/CaM. Format as ina–f. (h,j) C-lobe CDI at 300 ms, unchanged by NSCaTE mutations. Bars inj, mean±s.e.m. of ~5 cells. (i,k) Changes inKa,EFFof NSCaTE module for Ca2+/CaM12via 33-FRET. Each symbol ini, mean±s.e.m. of ~5 cells. (l) C-lobeCDIversusKa,EFFdeviates from Langmuir, as inFig. 2c. Figure 4: iTL analysis of Ca 2+ /CaM effector role of NSCaTE module of Ca V 1.3 channels. ( a ) Cartoon depicting NSCaTE as putative effector interface for N-lobe of Ca 2+ /CaM. ( b ) Exemplar Ca V 1.3 whole-cell currents exhibiting robust isolated N-lobe CDI, as seen from the rapid decay of Ca 2+ current (black trace). Corresponding stick-figure subsystem appears on the left. W[44]A mutation abolishes N-lobe CDI, as seen from the lack of appreciable Ca 2+ current decay (red trace). Gray trace, averaged Ba 2+ trace for WT and W[44]A constructs. Horizontal scale bar, 100 ms; vertical scale bar, 0.2 nA Ca 2+ current (red, W44A; black, WT). ( c ) FRET two-hybrid binding curves for Ca 2+ /CaM 34 and NSCaTE segment, with FRET partners schematized on the left. WT pairing in black; W[44]A mutant pairing in red. Each symbol, mean±s.e.m. of ~5 cells. ( d ) Bar-graph summary of N-lobe CDI for NSCaTE mutations measured after 800 ms depolarization, with NSCaTE sequence at the top, as numbered by position within Ca V 1.3. Data for W[44]A in red; dashed green line, WT. Bars, mean±s.e.m. of ~5 cells. ( e ) Association constants ( K a,EFF =1/ K d,EFF ) for Ca 2+ /CaM 34 binding to NSCaTE module evaluated for constructs exhibiting significant effects in panel d . Error bars, non-linear s.d. estimates. Data for W[44]A in red; dashed green line, WT. ( f ) Plotting N-lobe CDI versus K a,EFF uncovers a Langmuir, identifying NSCaTE as functionally relevant effector site. W[44]A in red; WT in green. ( g – l ) iTL fails to uphold NSCaTE as effector site for C-lobe of Ca 2+ /CaM. Format as in a – f . ( h , j ) C-lobe CDI at 300 ms, unchanged by NSCaTE mutations. Bars in j , mean±s.e.m. of ~5 cells. ( i , k ) Changes in K a,EFF of NSCaTE module for Ca 2+ /CaM 12 via 3 3 -FRET. Each symbol in i , mean±s.e.m. of ~5 cells. ( l ) C-lobe CDI versus K a,EFF deviates from Langmuir, as in Fig. 2c . Full size image Identification of the C-lobe Ca 2+ /CaM effector interface Satisfied by proof-of-principle tests of the iTL approach, we turned to identification of the as-yet-unknown effector site for the C-lobe form of CDI. Our screen focused upon the entire carboxy tail of Ca V 1.3 channels upstream of the IQ domain ( Fig. 5a , proximal Ca 2+ - i nactivation (PCI) domain), because switching these C-terminal segments in chimeric channels sharply influences this type of CDI [31] , [43] . For completeness, we initially characterized isolated N-lobe CDI for mutations throughout the PCI and found no appreciable decrement from WT levels ( Fig. 5b and Supplementary Note S12 ) as expected. Gaps indicate non-expressing configurations. By contrast, for isolated C-lobe CDI, the sharp diminution of CDI upon LGF→AAA substitution ( Fig. 5c , red) exemplifies just one of many newly discovered ‘hotspot’ loci residing in the PCI midsection ( Fig. 5f , rose and red; Supplementary Note S12 ). As a prelude to iTL analysis, we determined the binding of Ca 2+ /CaM to the PCI element ( Fig. 5g , left cartoon), and indeed the LGF substitution weakens interaction affinity ( Fig. 5d ). Likewise, binding of the isolated C-lobe of Ca 2+ /CaM to PCI was similarly attenuated by the LGF mutation ( Supplementary Note S11 ), arguing explicitly for disruption of a C-lobe interface. In addition, for loci demonstrating the strongest reduction in C-lobe CDI ( Fig. 5f , rose and red), corresponding Ca 2+ /CaM affinities were determined to also attenuate K a,EFF ( Fig. 5g and Supplementary Notes S11 and S12 ). Importantly, graphing C-lobe CDI versus binding affinity strikingly resolves a Langmuir relation ( Fig. 5i ), furnishing compelling evidence that the PCI midsection comprises an effector interface for the C-lobe of Ca 2+ /CaM. The green symbol corresponds to WT, and the red datum to the LGF mutant. Supplementary Note S1 specifically formulates equation 1 for this case. As expected, plots of N-lobe CDI versus binding affinity deviate from a Langmuir ( Fig. 5h ), much as in Fig. 2c . Overall, the impressive mirror-like inversion of results for NSCaTE ( Fig. 4f ) and PCI ( Fig. 5h ) underscores the considerable ability of iTL analysis to distinguish between effector sites of respective N- and C-lobe CDI. 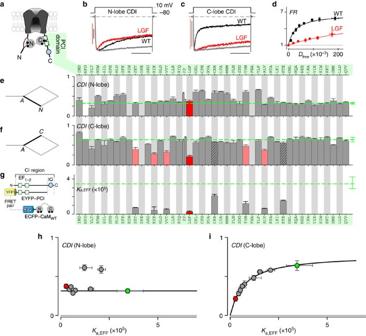Figure 5: iTL analysis of PCI segment as C-lobe Ca2+/CaM effector interface. (a) Channel cartoon depicting PCI segment as putative effector site for C-lobe of Ca2+/CaM. (b) Isolated N-lobe CDI for WT and LGF→AAA (LGF) mutant channels. Ca2+current for WT in red, and for LGF in red. Gray, averaged Ba2+trace. Horizontal scale bar, 100 ms; vertical scale bar, 0.2 nA Ca2+current (red, LGF; black, WT). (c) Isolated C-lobe CDI for WT and LGF mutant channels, indicating strong CDI attenuation by LGF mutation. Format as inb. (d) FRET two-hybrid binding curves for Ca2+/CaM pitted against PCI segments, for WT (black) and LGF (red). Each symbol, mean±s.e.m. from~9 cells. (e) Bar-graph summary confirming no appreciable reduction of isolated N-lobe CDI, over all alanine scanning mutants across the PCI region (sequence at the top). Schematic of corresponding system under investigation at the left. Green dashed line, WT; red, LGF mutant; gaps, non-expressing configurations. Bars, mean±s.e.m. of ~5 cells. (f) Bar-graph summary, C-lobeCDIfor alanine scan of PCI. Red bar, LGF→AAA mutant showing strong CDI reduction. Rose bar, other loci showing substantial CDI reduction. Hashed, randomly chosen loci for subsequent FRET analysis below. Bars, mean±s.e.m. of ~5 cells. (e,f) CDI decrease for YLT cluster (Fig. 5e) reflects reduced Ca2+entry from 30 mV depolarizing shift in activation, not CDI attenuationper se. Shifts for all other loci were at most ±10 mV (not shown). (g) Association constants for Ca2+/CaM binding to PCI region, with FRET partners as diagrammed on the left. Green dashed line, WT profile. PCI mutations yielding large C-lobeCDIdeficits were chosen for FRET analysis (red and rose inf), as well as those chosen at random (hashed inf). Error bars, nonlinear estimates of standard deviation. (h) Plots of N-lobe CDI versusKa,EFFfor Ca2+/CaM binding to PCI deviated from Langmuir. Red, LGF; green, WT. (i) Alternatively, plotting C-lobe CDI revealed Langmuir relation, supporting PCI as C-lobe Ca2+/CaM effector site. Symbols as inh. Figure 5: iTL analysis of PCI segment as C-lobe Ca 2+ /CaM effector interface. ( a ) Channel cartoon depicting PCI segment as putative effector site for C-lobe of Ca 2+ /CaM. ( b ) Isolated N-lobe CDI for WT and LGF→AAA (LGF) mutant channels. Ca 2+ current for WT in red, and for LGF in red. Gray, averaged Ba 2+ trace. Horizontal scale bar, 100 ms; vertical scale bar, 0.2 nA Ca 2+ current (red, LGF; black, WT). ( c ) Isolated C-lobe CDI for WT and LGF mutant channels, indicating strong CDI attenuation by LGF mutation. Format as in b . ( d ) FRET two-hybrid binding curves for Ca 2+ /CaM pitted against PCI segments, for WT (black) and LGF (red). Each symbol, mean±s.e.m. from~9 cells. ( e ) Bar-graph summary confirming no appreciable reduction of isolated N-lobe CDI, over all alanine scanning mutants across the PCI region (sequence at the top). Schematic of corresponding system under investigation at the left. Green dashed line, WT; red, LGF mutant; gaps, non-expressing configurations. Bars, mean±s.e.m. of ~5 cells. ( f ) Bar-graph summary, C-lobe CDI for alanine scan of PCI. Red bar, LGF→AAA mutant showing strong CDI reduction. Rose bar, other loci showing substantial CDI reduction. Hashed, randomly chosen loci for subsequent FRET analysis below. Bars, mean±s.e.m. of ~5 cells. ( e , f ) CDI decrease for YLT cluster ( Fig. 5e ) reflects reduced Ca 2+ entry from 30 mV depolarizing shift in activation, not CDI attenuation per se . Shifts for all other loci were at most ±10 mV (not shown). ( g ) Association constants for Ca 2+ /CaM binding to PCI region, with FRET partners as diagrammed on the left. Green dashed line, WT profile. PCI mutations yielding large C-lobe CDI deficits were chosen for FRET analysis (red and rose in f ), as well as those chosen at random (hashed in f ). Error bars, nonlinear estimates of standard deviation. ( h ) Plots of N-lobe CDI versus K a,EFF for Ca 2+ /CaM binding to PCI deviated from Langmuir. Red, LGF; green, WT. ( i ) Alternatively, plotting C-lobe CDI revealed Langmuir relation, supporting PCI as C-lobe Ca 2+ /CaM effector site. Symbols as in h . Full size image C-lobe CDI also requires IQ domain interaction with the PCI element Though the IQ domain alone does not appear to be an effector site for Ca 2+ /CaM ( Fig. 3 ), alanine substitutions in this element nonetheless attenuated the C-lobe CDI [7] , [10] , [11] , [28] , [31] , a result reproduced for reference in Fig. 6a . Might the departure of Ca 2+ /CaM to NSCaTE ( Fig. 4 ) and PCI elements ( Fig. 5 ) then allow the IQ domain to rebind elsewhere, in a manner also required for C-lobe CDI? Thus viewed, IQ-domain mutations could diminish C-lobe CDI by weakening this rebinding, but in a way that correlates poorly with IQ-peptide binding to Ca 2+ /CaM in isolation. As C-lobe CDI can be conferred to Ca V 2 channels by substituting PCI and IQ elements from Ca V 1 [31] , [43] , will the requisite rebinding involve association between these very elements? 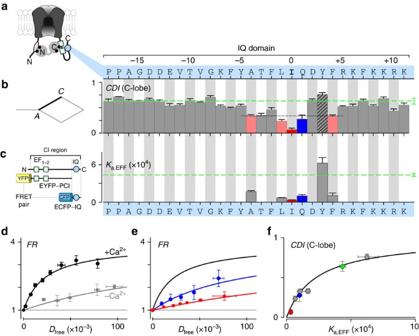Figure 6: Role of IQ domain in C-lobe CDI. (a) Cartoon depicting putative binding interaction between IQ domain and PCI segment, which is also required for C-lobe CDI. (b) Bar-graph summary of C-lobe CDI measured for alanine scan of IQ domain, reproduced fromFig. 3b. Strongest CDI reduction for I[0]A mutant (red), followed closely by loci affiliated with rose and blue bars underneath black dashed line. Dashed green line, WT. (c) Association constantsKa,EFFdetermined for 33-FRET binding between IQ domain and PCI region (partners diagrammed at left), under elevated levels of Ca2+. WT profile, green dashed line. Bars,Ka,EFFfor mutants with strongest effects (colored bars inb) or chosen at random (hashed bars inb). Error bars, nonlinear s.d. estimates. (d) Exemplar 33-FRET binding curves for IQ/PCI interaction. Each symbol, mean±s.e.m. of ~8 cells. Absent Ca2+, the IQ domain associates only weakly with the PCI region (gray). However, elevated Ca2+greatly enhances binding (black). (e) 33-FRET binding curves for I[0]A (red) and Q[1]A (blue) mutations under elevated Ca2+. Each symbol, mean±s.e.m. of ~5 cells. Fit for WT IQ/PCI interaction reproduced fromdin black. (f) Plotting C-lobe CDI versusKa,EFFunder elevated Ca2+unveils a well-resolved Langmuir relation. WT (green), I[0]A (red), and Q[1]A (blue). Figure 6: Role of IQ domain in C-lobe CDI. ( a ) Cartoon depicting putative binding interaction between IQ domain and PCI segment, which is also required for C-lobe CDI. ( b ) Bar-graph summary of C-lobe CDI measured for alanine scan of IQ domain, reproduced from Fig. 3b . Strongest CDI reduction for I[0]A mutant (red), followed closely by loci affiliated with rose and blue bars underneath black dashed line. Dashed green line, WT. ( c ) Association constants K a,EFF determined for 3 3 -FRET binding between IQ domain and PCI region (partners diagrammed at left), under elevated levels of Ca 2+ . WT profile, green dashed line. Bars, K a,EFF for mutants with strongest effects (colored bars in b ) or chosen at random (hashed bars in b ). Error bars, nonlinear s.d. estimates. ( d ) Exemplar 3 3 -FRET binding curves for IQ/PCI interaction. Each symbol, mean±s.e.m. of ~8 cells. Absent Ca 2+ , the IQ domain associates only weakly with the PCI region (gray). However, elevated Ca 2+ greatly enhances binding (black). ( e ) 3 3 -FRET binding curves for I[0]A (red) and Q[1]A (blue) mutations under elevated Ca 2+ . Each symbol, mean±s.e.m. of ~5 cells. Fit for WT IQ/PCI interaction reproduced from d in black. ( f ) Plotting C-lobe CDI versus K a,EFF under elevated Ca 2+ unveils a well-resolved Langmuir relation. WT (green), I[0]A (red), and Q[1]A (blue). Full size image Initially disappointing was the existence of only low-affinity binding between IQ and PCI modules ( Fig. 6c , left cartoon; Fig. 6d , gray) under conditions of resting intracellular calcium [3] . By contrast, under elevated Ca 2+ , robust interaction between the same IQ/PCI FRET pair was observed, with K a-PCI–IQ =4.35 × 10 −5 D free units −1 ( Fig. 6d , black). In fact, this Ca 2+ -dependent interaction accords well with a role in triggering CDI, and likely arises from a requirement for Ca 2+ /CaM to bind the PCI domain before appreciable IQ association occurs ( Supplementary Note S13 ). Beyond mere binding, however, functionally relevant interaction would be decreased by the same IQ-domain mutations that reduced C-lobe CDI. In this regard, IQ peptides bearing I[0]A or Q[1]A substitutions actually demonstrated strong and graded reductions in affinity ( Fig. 6e , respective red and blue symbols), coarsely matching observed deficits in C-lobe CDI ( Fig. 6b ). Figure 6c summarizes the results of these and other FRET-binding assays ( Supplementary Note S14 ) performed for loci with the strongest effects on C-lobe CDI ( Fig. 6b , coloured bars under dashed black threshold). With these data, quantitative iTL analysis could be undertaken, where the presumed CDI transition in question would be the γ 2 transduction step in Fig. 2a , and the relevant form of equation 1 is specified in Supplementary Note S15 . Remarkably, plotting C-lobe CDI ( Fig. 6b ) versus IQ/PCI-binding affinity ( Fig. 6c ) indeed resolves a Langmuir ( Fig. 6f ). Thus, C-lobe CDI likely requires a tripartite complex of IQ, PCI, and C-lobe Ca 2+ /CaM ( Fig. 6a ). ApoCaM preassociation within the PCI domain Having explored Ca 2+ /CaM, we turned to apoCaM interactions. Elsewhere [42] we have shown that apoCaM preassociates with a surface that at least includes [2] , [4] , [5] , [20] the IQ element. Furthermore, homology modelling [42] of a related apoCaM/IQ structure for Na V channels [44] , [45] suggests that the Ca V 1.3 IQ module interacts with the C-lobe of apoCaM. Will the N-lobe of apoCaM then bind the PCI domain ( Fig. 7a )? If so, then our earlier PCI mutations could have weakened N-lobe apoCaM interaction, and potentially diminished CDI by favouring configuration E channels ( Fig. 1a , incapable of inactivation). This effect would not have been apparent thus far, as we invariably overexpressed CaM. However, with only endogenous CaM present in Fig. 7e , CDI reflects the operation of a system that includes configuration E (left schematic), and the observed CDI CaMendo is indeed strongly attenuated by mutations at many loci (rose and red bars). 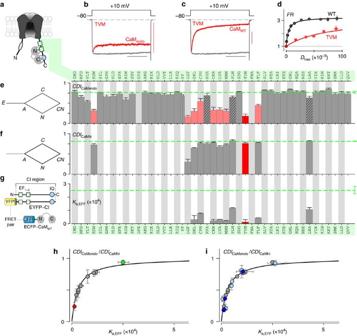Figure 7: Footprint of apoCaM preassociation with the PCI segment. (a) Channel cartoon depicting apoCaM preassociated with the CI region, with C-lobe engaging IQ domain, and N-lobe associated with PCI region. (b) Whole-cell currents for TVM→AAA mutant in the PCI segment (Ca2+in red; Ba2+in gray), with only endogenous CaM present. Horizontal scale bar, 100 ms; vertical scale bar, 0.2 nA Ca2+current. (c) Overexpressing CaMWTrescues CDI for TVM→AAA mutation, suggesting that PCI region harbours an apoCaM preassociation locus. Format as inb. (d) 33-FRET binding curves show strong apoCaM binding to CI region. WT in black; TVM→AAA in red. Each symbol, mean±s.e.m. of ~7 cells. (e) Bar-graph summary of CDI with only endogenous CaM present (CDICaMendo), across alanine scan of PCI region. TVM→AAA (red) shows strongest effect, with rose colored bars also showing appreciable CDI reduction. Bars, mean±s.e.m. of ~5 cells. Left, schematic of relevant CaM subsystem. (f) Bar-graph summary of CDI rescue upon overexpressing CaMWT(CDICaMhi), for mutations showing significant loss of CDI (coloured bars ine), or chosen at random (hashed bars ine). Bars, mean±s.e.m. of ~5 cells. Corresponding subsystem of regulation on the left. (g) Bar-graph summary ofKa,EFFfor apoCaM binding to CI region, with partners as sketched on the left. Data obtained for nearly all mutants with significant CDI reduction (coloured ine), and for some mutants chosen at random (hashed ine). Error bars, non-linear estimates of s.d. (h) iTL analysis confirms role of PCI as functionally relevant apoCaM site. PlottingCDICaMendo/CDICaMhi(e,f) versusKa,EFFfor apoCaM/CI binding uncovers well-resolved Langmuir relation. TVM→AAA, red; WT, green. (i) Overlaying like data for IQ-domain analysis presented elsewhere42(blue symbols here) displays remarkable agreement, consistent with the same apoCaM binding both PCI and IQ domains. Deep blue symbols, A[−4], I[0], F[+4] hotspots for apoCaM interaction with IQ element. Figure 7: Footprint of apoCaM preassociation with the PCI segment. ( a ) Channel cartoon depicting apoCaM preassociated with the CI region, with C-lobe engaging IQ domain, and N-lobe associated with PCI region. ( b ) Whole-cell currents for TVM→AAA mutant in the PCI segment (Ca 2+ in red; Ba 2+ in gray), with only endogenous CaM present. Horizontal scale bar, 100 ms; vertical scale bar, 0.2 nA Ca 2+ current. ( c ) Overexpressing CaM WT rescues CDI for TVM→AAA mutation, suggesting that PCI region harbours an apoCaM preassociation locus. Format as in b . ( d ) 3 3 -FRET binding curves show strong apoCaM binding to CI region. WT in black; TVM→AAA in red. Each symbol, mean±s.e.m. of ~7 cells. ( e ) Bar-graph summary of CDI with only endogenous CaM present ( CDI CaMendo ), across alanine scan of PCI region. TVM→AAA (red) shows strongest effect, with rose colored bars also showing appreciable CDI reduction. Bars, mean±s.e.m. of ~5 cells. Left, schematic of relevant CaM subsystem. ( f ) Bar-graph summary of CDI rescue upon overexpressing CaM WT ( CDI CaMhi ), for mutations showing significant loss of CDI (coloured bars in e ), or chosen at random (hashed bars in e ). Bars, mean±s.e.m. of ~5 cells. Corresponding subsystem of regulation on the left. ( g ) Bar-graph summary of K a,EFF for apoCaM binding to CI region, with partners as sketched on the left. Data obtained for nearly all mutants with significant CDI reduction (coloured in e ), and for some mutants chosen at random (hashed in e ). Error bars, non-linear estimates of s.d. ( h ) iTL analysis confirms role of PCI as functionally relevant apoCaM site. Plotting CDI CaMendo / CDI CaMhi ( e , f ) versus K a,EFF for apoCaM/CI binding uncovers well-resolved Langmuir relation. TVM→AAA, red; WT, green. ( i ) Overlaying like data for IQ-domain analysis presented elsewhere [42] (blue symbols here) displays remarkable agreement, consistent with the same apoCaM binding both PCI and IQ domains. Deep blue symbols, A[−4], I[0], F[+4] hotspots for apoCaM interaction with IQ element. Full size image We tested for decreased preassociation as the basis of this effect, by checking whether CDI resurged upon strongly overexpressing CaM WT . This manoeuvre should act via mass action to eliminate CaM-less channels [20] , restrict channels to the subsystem on the left of Fig. 7f and restore CDI. For all loci demonstrating appreciable reduction of CDI CaMendo ( Fig. 7e , rose and red), CDI was measured under strongly overexpressed CaM WT ( CDI CaMhi ), as summarized in Fig. 7f . As the baseline, we confirmed that elevating CaM WT hardly affected CDI of WT channels (compare WT, dashed green lines in Fig. 7e ). The high apoCaM affinity of WT channels renders configuration E channels rare, even with only endogenous apoCaM present [20] . By contrast, the TVM mutant exhibits an impressive return of CDI upon elevating CaM WT ( Fig. 7b ), as do many other mutants ( Fig. 7f and Supplementary Note S16 ). Critically, scrutiny of the underlying configurations ( Fig. 7e , left) reveals that CDI CaMendo = CDI CaMhi × F b , where F b is the fraction of channels prebound to apoCaM with only endogenous CaM present. This relation holds true, even with a residual CDI CaMhi shortfall compared with WT (for example, Fig. 7f , LGF). This is so, because a CDI CaMhi deficit mirrors changes in the diamond subsystem of Fig. 7f (left), which are identically present in CDI CaMendo measurements ( Fig. 7e ). Thus aware, we tested whether apoCaM binding to the entire CI domain (spanning IQ and PCI modules) mirrors resurgent CDI ( Fig. 7g , left cartoon; Supplementary Note S17 ). The WT pairing showed robust interaction with K a,EFF =2.5 × 10 −4 D free units −1 ( Fig. 7d , black; Fig. 7g , green dashed line). By contrast, the TVM pairing, corresponding to strong resurgent CDI ( Fig. 7b ), exhibited far weaker affinity ( Fig. 7d , red; K a,EFF =0.13 × 10 −4 D free units −1 ). Figure 7g tallies the graded decrease of K a,EFF for these and other pairings ( Supplementary Note S16 ). Most rigorously, if PCI contacts indeed mediate apoCaM preassociation, then plotting CDI CaMendo / CDI CaMhi (= F b ) versus the K a,EFF for apoCaM/CI interaction ( Fig. 7g ) should decorate a Langmuir relation ( Supplementary Note S18 ). Indeed, just such a relation ( Fig. 7h ) is resolved ( Fig. 7e–g ), arguing that the N-lobe of apoCaM interfaces with corresponding PCI loci. Notably, this relation is identical to that reported elsewhere for IQ mutations on the same CI module [42] . Figure 7i explicitly overlays PCI and IQ data (in blue), and this striking resolution of a single Langmuir accords with one and the same apoCaM binding PCI and IQ domains. These experiments fundamentally transform the prevailing molecular view of CaM regulation of Ca 2+ channels. The field has long been dominated by an IQ-centric scheme [2] , [5] , [7] , [9] , [10] , [25] , [28] , wherein indwelling apoCaM begins preassociated with a C-terminal IQ domain, and remains bound to this element upon CaM interaction with Ca 2+ . Here our new proposal establishes substantial exchange of CaM to alternate effector loci ( Fig. 8a ). ApoCaM preassociates with an interface that includes, but is not limited to, the IQ domain (configuration A ): the C-lobe binds the IQ (cyan circle) and the N-lobe binds the central midsection of the PCI (green box). Ca 2+ binding to the N-lobe yields configuration I N , wherein this lobe binds the NSCaTE module on the channel N terminus (pink oval) to trigger the N-lobe CDI. Ensuing Ca 2+ binding to the C-lobe induces configuration I CN , with C-lobe binding the proximal PCI midsection (green square) and IQ engagement [25] . If Ca 2+ only binds the C-lobe, the system adopts configuration I C , corresponding to C-lobe CDI. Ultimately, Ca 2+ /CaM exchange to effector loci diminishes opening, perhaps via allosteric coupling of carboxy-tail conformation to a contiguous IVS6 segment implicated in activation [46] , [47] and inactivation [48] . Only a single CaM is present [22] , [23] ( Supplementary Note S17 ). 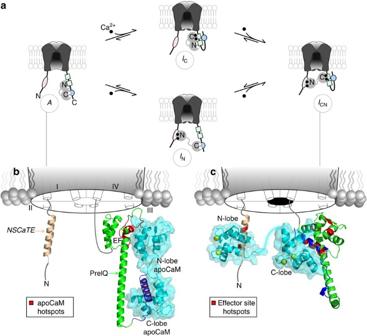Figure 8: New view of CaM regulatory configurations of CaV1.3 channels. (a) Molecular layout of configurationsA,IC,INandICNfor conceptual scheme inFig. 1a. ApoCaM preassociates with CI region: C-lobe articulates IQ domain, and N-lobe engages the PCI segment. Once Ca2+binds CaM, the N-lobe of Ca2+/CaM departs to NSCaTE on channel N terminus, eliciting N-lobe CDI (IN). Alternatively, the C-lobe of Ca2+/CaM migrates to PCI segment, recruiting IQ domain to tripartite complex (IC). Finally,ICNcorresponds to channel that has undergone both N- and C-lobe CDI. (b)De novomodel of CaV1.3 CI region docked to apoCaM (PCI region: green; IQ domain: blue). ApoCaM hotspots (Fig. 6e–g) in red. C-lobe of apoCaM contacts IQ, whereas N-lobe binds EF-hand region. (c) Left, atomic structure of NSCaTE bound to N-lobe of Ca2+/CaM (2LQC33). NSCaTE peptide in tan; and N-lobe Ca2+/CaM in cyan. Ca2+, yellow. N-lobe CDI hotspots on NSCaTE in red. Right,de novomodel of tripartite IQ-PCI-Ca2+/CaM complex (PCI region, green; IQ domain, blue). C-lobe CDI hotspots in red for both PCI and IQ domains. Figure 8: New view of CaM regulatory configurations of Ca V 1.3 channels. ( a ) Molecular layout of configurations A , I C , I N and I CN for conceptual scheme in Fig. 1a . ApoCaM preassociates with CI region: C-lobe articulates IQ domain, and N-lobe engages the PCI segment. Once Ca 2+ binds CaM, the N-lobe of Ca 2+ /CaM departs to NSCaTE on channel N terminus, eliciting N-lobe CDI ( I N ). Alternatively, the C-lobe of Ca 2+ /CaM migrates to PCI segment, recruiting IQ domain to tripartite complex ( I C ). Finally, I CN corresponds to channel that has undergone both N- and C-lobe CDI. ( b ) De novo model of Ca V 1.3 CI region docked to apoCaM (PCI region: green; IQ domain: blue). ApoCaM hotspots ( Fig. 6e–g ) in red. C-lobe of apoCaM contacts IQ, whereas N-lobe binds EF-hand region. ( c ) Left, atomic structure of NSCaTE bound to N-lobe of Ca 2+ /CaM (2LQC [33] ). NSCaTE peptide in tan; and N-lobe Ca 2+ /CaM in cyan. Ca 2+ , yellow. N-lobe CDI hotspots on NSCaTE in red. Right, de novo model of tripartite IQ-PCI-Ca 2+ /CaM complex (PCI region, green; IQ domain, blue). C-lobe CDI hotspots in red for both PCI and IQ domains. Full size image The structures of many of these configurations are presently unknown, but ab initio and homology modelling here confirms the plausibility of these configurations. Concerning the apoCaM/channel complex, Fig. 8b displays a homology model of the C-lobe complexed with the IQ domain [42] (blue), based on an analogous atomic structure from Na V channels [44] , [45] . Key IQ-domain hotspots for apoCaM preassociation (red) are rationalized by this model [42] . To portray the N-lobe as shown in Fig. 8b , we utilized ab initio structural prediction of the CI domain with the Rosetta package [49] ( Supplementary Note S19 ), yielding a PCI domain (green) with two vestigial EF hands, and a protruding helix (‘preIQ’ subelement). The EF-hand module (EF) resembles the structure of a homologous segment of Na V channels [50] , [51] , and a helical segment has been resolved in atomic structures of analogous Ca V 1.2 segments [36] , [37] . Reassuringly, N-lobe apoCaM hotspots adorn the surface of this PCI model (red coloration), within the more C-terminal of the two EF hands. Accordingly, we appose the atomic structure of the N-lobe (1 CFD) to this segment of the PCI model, initially using a shape-complementarity docking algorithm [52] ( PatchDock ), followed by refinement with docking protocols of Rosetta ( Supplementary Note S20 ). Of note, the configuration of the N-lobe explains the outright enhancement of N-lobe CDI by PCI mutations in the region of putative N-lobe contact (compare Figs 5e and 7e , GKL through TLF). Weakening channel binding to the N-lobe ( Fig. 2a , state 1) would, through connection to other states, increase state 5 occupancy, thereby boosting N-lobe CDI ( Supplementary Note S21 ). By contrast, no N-lobe CDI enhancement was observed for IQ substitutions at the central isoleucine (I[0]) and downstream [42] , consistent with IQ binding the C-lobe of apoCaM. Figure 8c displays a model of Ca 2+ /CaM complexed with the channel. The N-lobe bound to NSCaTE is an NMR structure [33] , and functional N-lobe CDI hotspots correspond well with intimate contact points (red). C-lobe CDI hotspots also adorn the surface of the upstream EF-hand region of an alternative ab initio model of the PCI ( Fig. 8c , red; Supplementary Note S19 ). The IQ domain and atomic structure of the C-lobe of Ca 2+ /CaM (3BXL) were then computationally docked ( Supplementary Note S22 ), yielding a rather canonical CaM/peptide complex where the channel contributes a surrogate lobe of CaM. Overall, this framework promises to set the table for future structural biology and structure–function work. More broadly, this regulatory scheme may explain paradoxes and open horizons. First, it has been asked how Ca 2+ /CaM could ever leave the IQ domain, when the binding affinity between these elements is so high [4] , [5] , [29] , [39] , [53] (for example, K a/CaM–IQ =5.88 × 10 −4 D free −1 units in Fig. 3c ). The answer may arise from the competing binding affinity for the tripartite complex ( Fig. 8a , I CN ), which multivalent ligand binding theory [54] would approximate as K a/CaM–PCI–IQ ~ K a/CaM–PCI × K a/PCI-IQ × (local concentration of IQ)=(4.35 × 10 −5 D free units −1 ) × (3.45 × 10 −5 D free units −1 ) × (1.36 × 10 8 D free units)~0.2 D free units −1 , a value far larger than K a/CaM–IQ ( Supplementary Note S23 ). Second, our scheme offers new interfaces targetable by native modulators and drug discovery. As L-type channel CDI influences cardiac arrhythmogenic potential [15] , [18] and Ca 2+ load in substantia nigral neurons prone to degeneration in Parkinson’s [55] , one could envisage a screen for selective modulators of N- or C-lobe CDI [19] . Third, our results offer a fine-grained roadmap for Ca V 1-2 splice/editing variants and channelopathies [56] . Indeed, we suspect that the design principles revealed here may generalize widely to other molecules modulated by CaM [45] , [50] , [51] , [57] . Molecular biology To simplify mutagenesis, the WT construct in this study was an engineered Ca V 1.3 construct α 1DΔ1626 , nearly identical to and derived from the native rat brain variant ( α 1D , AF3070009). Briefly, the α 1DΔ1626 construct, as contained with mammalian expression plasmid pCDNA6 (Invitrogen), features introduction of a silent and unique Kpn I site at a position corresponding to ~50 amino acid residues upstream of the C-terminal IQ domain (G 1538 T 1539 ). As well, a unique Bgl II restriction site is present at a locus corresponding to ~450 amino acid residues upstream of the IQ domain. Finally, a unique Xba I and stop codon have been engineered to occur immediately after the IQ domain. These attributes accelerated construction of cDNAs encoding triple alanine mutations of α 1DΔ1626 . Point mutations of channel segments were made via QuikChange mutagenesis (Agilent) before PCR amplification and insertion into the full-length α 1DΔ1626 channel construct via restriction sites Bgl II/ Kpn I, Kpn I/ Xba I or Bgl II/ Xba I. Some triple alanine mutation constructs included a seven amino acid extension (SRGPAVRR) after residue 1626. For FRET two-hybrid constructs, fluorophore-tagged (all based on enhanced cyan fluorescent protein (ECFP) and enhanced yellow fluorescent protein (EYFP)) CaM constructs were made as described [4] . Other FRET constructs were made by replacing CaM with appropriate PCR-amplified segments, via unique Not I and Xba I sites flanking CaM [4] . YFP–CaM C ( Supplementary Fig. S10 ) was YFP fused to the C-lobe of CaM (residues 78–149). To aid cloning, the YFP-tagged CI region was made with a 12 residue extension (SRGPYSIVSPKC) via Not I/ Xba I sites as above. This linker did not alter apoCaM binding affinity versus WT YFP-tagged CI region (not shown). Throughout, all segments subject to PCR or QuikChange mutagenesis were verified in their entirety by sequencing. Transfection of HEK293 cells For whole-cell patch clamp experiments, HEK293 cells were cultured on 10-cm plates, and channels transiently transfected by a calcium phosphate method [9] . We applied 8 μg of complementary DNA encoding the desired channel α 1 -subunit, along with 8 μg of rat brain β 2a (M80545) and 8 μg of rat brain α 2 δ (NM012919.2) subunits. We utilized the β 2a auxiliary subunit to minimize voltage-dependent inactivation. For experiments involving CaM overexpression, we coexpressed 8 μg of rat CaM WT , CaM 12 or CaM 34 , as described [9] . All of the above cDNA constructs were included within mammalian expression plasmids with a cytomegalovirus promoter. To boost expression, cDNA for simian virus 40T antigen (1–2 μg) was cotransfected. For FRET two-hybrid experiments, HEK293 cells were cultured on glass-bottom dishes and transfected with FuGENE 6 (Roche) before epifluorescence microscope imaging [4] . Electrophysiology/FRET experiments were performed at room temperature 1–3 days after transfection. Whole-cell recording Whole-cell recordings were obtained using an Axopatch 200 A amplifier (Axon Instruments). Electrodes were made from borosilicate glass capillaries (World Precision Instruments, MTW 150-F4) yielding 1–3 MΩ resistances, which were in turn compensated for series resistance by >70%. Currents were low-pass filtered at 2 kHz before digital acquisition at several times that frequency. A P/8 leak-subtraction protocol was used. The internal solution contained (in mM): CsMeSO 3 , 114; CsCl, 5; MgCl 2 , 1; MgATP, 4; HEPES (pH 7.4), 10; and BAPTA (1,2-bis( o -aminophenoxy)ethane- N,N,N′,N′ -tetraacetic acid), 10; at 290 mOsm adjusted with glucose. The bath solution was (in mM): TEA-MeSO 3 , 102; HEPES (pH 7.4), 10; CaCl 2 or BaCl 2 , 40; at 300 mOsm, adjusted with TEA-MeSO 3 . FRET optical imaging We conducted FRET two-hybrid experiments in HEK293 cells cultured on glass-bottom dishes, using an inverted fluorescence microscope as extensively described by our laboratory [4] . Experiments utilized a bath Tyrode’s solution containing either 2 mM Ca 2+ for experiments probing apoCaM binding or 10 mM Ca 2+ with 4 μM ionomycin (Sigma-Aldrich, MO) for elevated Ca 2+ experiments. The 3 3 -FRET efficiencies ( E A ) were computed as elaborated in our prior publications [4] . E-FRET efficiencies ( E D ), whose measurement methodology was developed and refined in other labortories [41] , could be determined from the same single-cell 3 3 -FRET measurements using the following relationship, which expresses E D in terms of our own calibration metrics and standard measurements: where G is a constant, defined as S FRET , S YFP and S CFP correspond to fluorescent measurements from the same cell using FRET, YFP and CFP cubes, whose spectral properties have been detailed previously [4] . R D1 and R A are constants relating to the respective spectral properties of ECFP and EYFP; ε CFP (440 nm)/ ε YFP (440 nm) approximates the ratio of molar extinction coefficients of ECFP and EYFP at 440 nm, respectively; and M A / M D is the ratio of optical gain factors and quantum yields pertaining to EYFP and ECFP, respectively. Detailed descriptions of these parameters and their determination appear in our prior publications [4] . For all FRET efficiencies, spurious FRET relating to unbound ECFP and EYFP moieties has been subtracted [13] . For 3 3 -FRET, spurious FRET is linearly proportional to the concentration of CFP molecules, and the experimentally determined slope was obtained from cells coexpressing ECFP and EYFP fluorophores. Similarly, for E-FRET, the spurious FRET is linearly proportional to the concentration of EYFP molecules. The slope for this relationship A E−FRET can be obtained from: The methods for FRET two-hybrid binding curves have been extensively described in previous publications [3] , [4] , [41] . Briefly, binding curves were determined by least-squared error minimization of data from multiple cells, utilizing a 1:1 binding model, with adjustment of parameters K d,EFF and maximal FRET efficiency at saturating donor concentrations. For a small number of interactions involving mutations that strongly disrupted binding, the maximal FRET efficiency was set equal to that of the corresponding WT interaction and K d,EFF varied to minimize errors. The s.d. error bounds on K d,EFF estimates were determined by Jacobian error matrix analysis [58] . Supplementary Note S24 characterizes our FRET two-hybrid constructs, specifying their precise sequence composition, and behaviour via western blot and confocal imaging analysis. Molecular modelling De novo structural prediction was performed using the Robetta online server [49] ( http://robetta.bakerlab.org ) as described in Supplementary Notes S19, S20–S22 . We used web-based molecular docking programs, PatchDock [52] ( http://bioinfo3d.cs.tau.ac.il/PatchDock/ ) and FireDock [59] ( http://bioinfo3d.cs.tau.ac.il/FireDock/ ) to obtain preliminary models for molecular docking. Such preliminary models were subsequently used as starting models for further structural modelling and refinement using a customized docking protocol of PyRosetta [60] . A homology model of the C-lobe of apoCaM bound to IQ domain was constructed as described elsewhere [42] . All molecular models and atomic structures were visualized and rendered using PyMOL v1.2r1. (DeLano Scientific, LLC). How to cite this article: Ben Johny, M. et al. Dynamic switching of calmodulin interactions underlies Ca 2+ regulation of Ca V 1.3 channels. Nat. Commun . 4:1717 doi: 10.1038/ncomms2727 (2013).